Creative arts and digitial interventions as potential tools in prevention and recovery from the mental health consequences of adverse childhood experiences 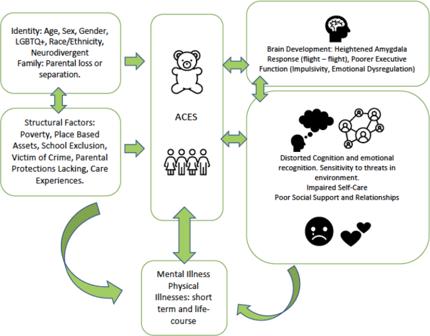Fig. 1: Pathways adversity to mental illness. Adverse Childhood experiences (ACES) affect young people from many demographic and social contexts (represented by the teddy bear) and involve adults/communities in terms of protections and therapeutic responses (i.e., structural factors). These two interact and the individual mechanisms affect families and communities. Adverse childhood experiences increase vulnerability for poor physical, mental and socio-educational outcomes throughout the lifespan [5] , [14] . Meta-analytic evidence suggests a dose-response effect, whereby exposure to four or more adverse experiences contributes to greater odds of poor health outcomes [16] . Data were pooled from 37 studies, indicating adverse experiences led to a 2–3 fold increase in the odds of smoking, heavy alcohol use, poor self-rated health, cancer, heart disease, and respiratory disease. There was also a 4–6 fold higher odds of risky sexual behaviour and a 7–8 fold greater odds of exposure to interpersonal violence as victim or perpetrator [16] . Associations have also been reported for mental health conditions, including major depressive disorder [14] ; anxiety disorders [14] and psychosis [17] . Efforts to explore the aetiological relationships between adverse childhood experiences and the wellbeing of survivors have focused on the timing and type of adversities. Emotional abuse appears to increase the incidence of depressive disorders more than physical abuse; by contrast, physical abuse is associated with increased incidence of problematic drug use more so than emotional abuse [18] . Furthermore, the timing of adversities differentially impacts on the development of psychopathology. Exposure earlier in life (ages 0–5) predicted more symptoms of anxiety and depression in adulthood, than exposure at older ages (ages 6–8); the latter better predicted adult behavioural problems (e.g. substance misuse) [19] . One explanation for the sensitivity of age of exposure to adversity and consequential impact on mental health comes from the neuroscience literature. Studies have shown that exposure to adversities is associated with a significant reduction in grey-matter volume in the primary visual cortex amongst those who were survivors of childhood sexual abuse [20] , and in the left anterior and posterior cingulate cortex and bilateral precuneus (regions involved in self- evaluation and self-awareness) amongst those who were exposed to emotional abuse [21] . These reductions contribute to the altered development of sensory systems which process and interpret stress in response to adversity. This may contribute to distorted perceptions, cognitions and emotional regulation abilities that are associated with many mental illnesses. A key mechanism for poor outcomes, is that adversities are implicated in the development of emotion dysregulation and biases in emotion recognition [5] . In comparison to peers who have not experienced adversities, individuals who have a history of adversities report lower levels of emotional understanding [22] and distorted perceptions and greater sensitivity to negative facial expressions associated with anger and fear [23] . This can impact on relationships and levels of social support and communications with teachers and employers, leading to more challenges in progressing in life. These emotional impacts in turn may contribute to the development of mental health disorders rooted in emotional disturbances (i.e. anxiety, depression and PTSD) [24] . Similarly adverse childhood experiences are related to cognitive deficits such as the maladaptive formation of cognitive attributional styles [25] , hypersensitivity to threat in ambiguous situations and distortions in social information processing [5] . For example, being repeatedly exposed to adversities may contribute to the development of maladaptive cognitive processing, whereby individuals internalise the belief that the consequences of adversities are fixed and stable, have only negative consequences, and are attributable to their own conduct and behaviours. These cognitive schema contribute to the development of psychopathology such as depression [26] . Thus, adversities in childhood can lead to multiple mental health conditions with including post-traumatic stress, depression, psychoses, and dissociative symptoms, and may be complicated by poor self-care, self-medication (alcohol and substance misuse), and efforts to seek help or avoid help given this would become a reminder of the traumatic events. The mechanisms (Fig. 1 ) include direct and indirect pathways, and inflammatory responses are implicated in partially mediating the impacts of adversity [5] , [27] . Although adversities affect people across ethnicity, race, neurodiversity and socioeconomic groups, the intersecting effects of such factors are cumulative drivers of increased vulnerabilities. The frequency, types and experiences of adversities are differentially distributed across these groups and associated with disproportionate burdens of trauma amongst some communities [28] . The risk of adversities is greater amongst those who come from low income or single-parent households, or reside in unsafe neighbourhoods and lack access to health care [15] . In one study, data from the USA suggests that Black and Latino youth were exposed to a greater risk of experiencing ACEs in comparisons to their white peers [29] . As children and families belonging to racial and ethnic minority groups are more likely to live in low-income neighbourhoods and experience greater socioeconomic difficulties [30] , the interconnected systems-wide effect of disadvantage may increase vulnerabilities to the effect of adverse childhood experiences on mental and physical health and dampen recovery [30] . Albeit limited, there is some evidence to suggest similar patterns of elevated risks amongst racial and ethnic minorities in the United Kingdom [31] . Incidence rates of childhood maltreatment are one and a half times greater amongst those from a Black minority community in comparison to those from a white community [31] . Incidence rates are five-fold greater amongst those from the most socioeconomically deprived backgrounds in comparison to those from the least deprived in the UK [31] . In addition, neurodiverse individuals with Autism Spectrum Disorder (ASD) and ADHD are more likely to have experienced multiple adverse childhood experiences (ACEs) than neurotypical peers [32] . Intersectional factors contribute to the high prevalence of adverse childhood experiences globally [4] . These intersectional factors should be considered in the design of interventions to reduce barriers in service use and therapeutic impacts. More experiential research is needed to move away from the traditional approach of exploring adversity from a universal perspective and move towards developing a more nuanced understanding of experiences in specific populations, carrying specific intersectional vulnerabilities. Creative arts such as music, dance, drama and visual arts, and arts-based therapies are emerging as important approaches in the treatment of childhood trauma. Arts based research and interventions permit gradual exploration of adverse experiences, where the creator exercises control over disclosure, and non-verbal disclosure or awareness grows, leading to narration at deeper levels so offering an ethical and safer process that is less likely to lead to distress or trigger traumatic symptoms [33] , [34] , [35] . Evidence suggests that arts-based interventions improve sense of achievement, self-confidence, self-esteem, social skills, conflict resolution, problem solving, relationships and sense of belonging amongst adolescents [35] . Equally, these creative activities have been successful in improving mental health. Studies have found amongst young people who have experienced sexual abuse, music therapy [36] and group art therapy [37] have been effective in reducing depression, anxiety and PTSD symptoms. It is hypothesised that the participatory and creativity elements of arts-based interventions can contribute to resilience and recovery in a number of ways. For example, art has been found to elicit narrative and facilitate exposure to traumatic cues in a non-threatening and non-invasive manner, this in turn allows for the vocalisation of affective states and reduction in depressive and anxious symptoms [37] . Arts-based interventions have also been shown to modulate emotional responses to environmental cues and affect mood, through influencing emotional expression and regulation. Using creative practices to express and deal with negative emotions has been found to foster self-esteem, positive relationships and skills for overcoming adversity [34] . In addition, the group settings that creative arts-based intervention are often engaged in have the additional benefit of facilitating trust and disclosure amongst the young people partaking. This can provide an opportunity for individuals to realise that they are not alone in their experiences, have a sense of belonging and find peer-support. Young people are often described as ‘digital natives’. This aptitude coupled with the ubiquitous nature of digital technologies (i.e. smart phones and wearables) in modern life, support the therapeutic shift to digital health interventions (DHIs) such as apps, and virtual reality environments. These can increase the accessibility and support available to vulnerable and hard to reach individuals. These advantages alongside anonymity, instant feedback and cost-effectiveness [38] , suggest that digital interventions have the potential to be more helpful and overcome barriers to service use. Furthermore, stigma, fears about confidentiality, shame, financial costs [39] all undermine help seeking; digital approaches may also address the limited numbers of skilled clinicians and therapists in rural areas or in countries with less health spend (low and middle income countries). Young people seek emotional and social support and more flexible help, which digital technology can offer [40] . Indeed, there is evidence that young people exposed to ACEs use digital media more often than other young people [41] . Digital interventions can be used to screen and monitor mental health symptoms, and overcome physical barriers that affect attendance and retention at care services [42] . Young people prefer Digital Health Interventions (DHIs) which include features such as videos, limited text, personalisation and the ability to connect with others [43] . Thus the shift to using DHIs to support young people exposed to trauma has the potential to be revolutionise care experiences. Digital intervention in the form of serious games may have a positive impact for young people internalising symptoms of mental health [44] . Augmented and virtual reality adapted games have been used and found to be helpful for health care design and delivery, in physical and mental health conditions [44] . Similarly, digital story telling has been implemented as a narrative intervention when working with survivors of trauma [45] . By integrating personalised digital images, text, audio narration, and music, digital story telling supports the processing, organising, and integrating of traumatic memories. New narratives are created where the trauma is disentangled from the associated negative thoughts, reminders and emotions. However, there is a dearth of research in this area and more is needed to determine effectiveness and optimisation and personalisation for implementation. Indeed, adding creative arts methods as content, or trying to replicate creative processes in digital design may add value. However, this again needs evaluation. Although these approaches show promise for providing therapeutic support to young people exposed to adversities [44] , there are some concerns. Firstly, the experiences of virtual realities are dependent on gathering patient experiences to ensure this ‘real-world knowledge’ is included in the design to better support the ability to use and feel connected with virtual environments. The accuracy of the representation of real-world factors in the virtual environment can affect the ability to transfer learnt skills back into real world situations. Secondly, through digitalising interventions for traumatic experiences, therapeutic mechanisms such as active listening, empathic understanding and exploration of personal stories may be lost. There may still be a need for supervision, guided use of such interventions, and support to transition from immersive therapeutic technologies, back into ordinary life. Thirdly, there are ethical concerns about triggering disturbing experiences without appropriate support by a clinician or therapist, thus highlighting the need to always take participant safety into consideration when working with vulnerable individuals. Lastly, it can be challenging to preserve sufficient personalisation options in the up scaling of interventions delivered via digital platforms. Public and patient involvement at the time of development and testing of digital designs for interventions, could help overcome some of these concerns. For example, including elements of supervised individual and community support and incorporating creative elements in the generating digital content, could offer some reassurance and safeguards. For some, personal therapeutic support may be the only mechanism by which recovery is possible, thus identifying for whom digital interventions may work and how is an important research priority. There is a growth in digital platforms for mental health, and increased attention to designing virtual realities for therapeutic purposes. In the UK this is ever more pertinent due to the increased pressures NHS service provisions experience when providing care to young people who have experienced trauma, and especially so in the current climate of COVID-19 and limited capacity in health systems [46] . Currently there is some evidence on the effectiveness of digital interventions for young people’s mental illness, but much more is needed. Further research will need to evaluate the implementation, effectiveness and cost-effectiveness of interventions for a range of mental disorders (e.g. ADHD, psychosis and eating disorders), and comorbidities which are more common following multiple adversities. The interventions will need to address and be responsive to a number of social contexts. We anticipate future research will produce and evaluative a taxonomy for digital mental health interventions for adverse childhood experiences. It is important to consider the mechanistic drivers of trauma related mental illness, and recovery processes. Arts-based interventions show promise for recovery from trauma due to the creative and interactive elements, and such processes may be designed into digital interventions. Indeed, digital interventions already contain much arts content, so the distinction may not be as clear cut. A number of ethical dilemmas need exploration alongside the intervention design and delivery. The approach we propose is to engage young people in the co-design and implementation of research on digital health interventions.